The covalent modifier Nedd8 is critical for the activation of Smurf1 ubiquitin ligase in tumorigenesis Neddylation, the covalent attachment of ubiquitin-like protein Nedd8, of the Cullin-RING E3 ligase family regulates their ubiquitylation activity. However, regulation of HECT ligases by neddylation has not been reported to date. Here we show that the C2-WW-HECT ligase Smurf1 is activated by neddylation. Smurf1 physically interacts with Nedd8 and Ubc12, forms a Nedd8-thioester intermediate, and then catalyses its own neddylation on multiple lysine residues. Intriguingly, this autoneddylation needs an active site at C426 in the HECT N-lobe. Neddylation of Smurf1 potently enhances ubiquitin E2 recruitment and augments the ubiquitin ligase activity of Smurf1. The regulatory role of neddylation is conserved in human Smurf1 and yeast Rsp5. Furthermore, in human colorectal cancers, the elevated expression of Smurf1, Nedd8, NAE1 and Ubc12 correlates with cancer progression and poor prognosis. These findings provide evidence that neddylation is important in HECT ubiquitin ligase activation and shed new light on the tumour-promoting role of Smurf1. E3 ubiquitin ligases are the final effectors of the enzyme cascade that controls protein ubiquitylation. These proteins are commonly divided into two classes: the scaffold-type and the thioester bond intermediate-type [1] , [2] . The former type of E3s usually contains a RING (Really Interesting New Gene) finger domain [1] , whereas the latter contains a HECT (Homologous to E6-AP C Terminus) domain [2] . HECT E3s contain an active cysteine that forms a thioester bond with ubiquitin before catalysing substrate ubiquitylation [2] . In contrast, RING E3s are scaffolds that recruit E2 to the substrate to facilitate the direct transfer of ubiquitin [1] . Cullin-RING ligases (CRLs) are the most prominent class of E3s and play a pivotal role in the regulation of immunity, development, cell signalling and cell cycle [3] , [4] . Modification of CRLs by the ubiquitin-like Nedd8 (neural precursor cell-expressed developmentally downregulated protein 8), called neddylation, has been demonstrated to be essential for their activation [1] , [5] . In addition, non-cullin proteins such as p53, EGFR, pVHL, ribosomal proteins, Parkin, E2F-1 and TGFβ II receptor have been shown to be neddylated as well [6] , [7] , [8] , [9] , [10] , [11] , [12] , [13] . Nedd8 is activated by an E1 enzyme (that is, the APPBP1/Uba3 heterodimer), transferred to an E2-conjugating enzyme (Ubc12/UBE2M or UBE2F), and subsequently targeted to substrates that are recognized by an E3 ligase [14] , [15] . Neddylation is essential for the viability of most model organisms, including fission yeast, worms, flies and mice [16] , [17] , [18] , [19] . Excessive neddylation has been proved to be involved in cancer development [20] . A potent and selective inhibitor of NAE (Nedd8-activating enzyme, the heterodimer consisting of APPBP1/NAE1 andUba3), named MLN4924, has been demonstrated to suppress the growth of human tumours and is being evaluated in phase II clinical trials [21] , [22] . MLN4924 disrupts CRL-mediated protein turnover, leading to apoptosis in tumour cells. To date, regulation of HECT ligases by neddylation has not been reported. Notably, in contrast with several hundreds of ubiquitin ligases, only <10 Nedd8 ligases have been identified. For example, Roc1/Rbx1 and Dcn1 function synergistically to promote Nedd8 transfer from Ubc12 to Cullins [23] , [24] . MDM2, c-Cbl and IAPs have also been demonstrated to function as Nedd8 ligases to promote ligation to non-Cullin proteins [6] , [7] , [13] , [25] . All of the characterized Nedd8 E3s belong to the scaffold-type. Whether a HECT ligase can function as the thioester intermediate-type neddylation ligase has not been defined. Smad ubiquitylation regulatory factor 1 (Smurf1), a C2-WW-HECT ubiquitin ligase, is crucial for a variety of processes including bone homeostasis [26] , embryogenesis [27] , [28] and viral autophagy [29] . Previous studies demonstrated that CKIP-1 and Cdh1 enhance Smurf1 activity by promoting Smurf1–substrate interaction and disrupting Smurf1 homodimers, respectively [30] , [31] . Both activators are required for the activation of Smurf1 and the suppression of bone formation. Smurf1 and its close homologue Smurf2 antagonize the TGF-β/BMP pathways through ubiquitin-mediated degradation of crucial components of these pathways. The structural studies have shown that the Smurf2 HECT domain has a suboptimal E2-binding pocket that is regulated by adaptor protein such as Smad7 for enhancing the E3 ligase activity [32] . So far, the regulatory mechanism of Smurf1 ligase activity remains to be fully understood. In this study, we found that neddylation is critical for the activation of Smurf1 ubiquitin ligase activity. Neddylation enhances the ubiquitin E2 binding to Smurf1. Surprisingly, Smurf1 functions as a thioester bond-type Nedd8 ligase to catalyse its own neddylation. In human colorectal cancer, deregulation of Smurf1 is associated with the cancer progression and poor prognosis. Elevated Smurf1 expression correlates with cancer progression To investigate the potential clinical relevance of Smurf1 in colorectal cancer, we evaluated colorectal cancer tissue samples and matched adjacent normal tissue samples from 336 human subjects. Immunohistochemical analysis revealed that Smurf1 expression was significantly upregulated in cancer tissues compared with adjacent tissues ( Fig. 1a ; Supplementary Fig. 1a ). To better understand the relevance of Smurf1 to cancer, we divided the samples into groups based on the stage of tumour development and studied the differences in Smurf1 expression among these groups. In general, Smurf1 expression was lower in low-TNM stage tumours and higher in high-TNM stage tumours ( Fig. 1b–f ; Supplementary Fig. 1b,c ). Smurf1 expression was also lower in smaller tumours and higher in larger tumours ( Supplementary Fig. 1b ). Importantly, a follow-up analysis of patient survival demonstrated that patients whose tumours had high Smurf1 levels had significantly poorer survival than those with low Smurf1 levels ( Fig. 1g ). To investigate whether Smurf1 is involved in tumour growth, endogenous Smurf1 was depleted in HCT116 colorectal cancer cells by RNA interference (RNAi) with two independent target sites ( Fig. 1h ). The depletion of Smurf1 dramatically inhibited cell proliferation in cultured cells ( Supplementary Fig. 1d ) and tumour growth in nude mice ( Fig. 1h and data not shown). These data indicate that Smurf1 promotes the progression of colorectal cancer. 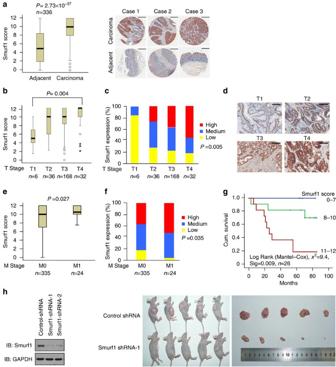Figure 1: Smurf1 expression is elevated in colorectal cancer tissues. (a) Smurf1 expression scores are shown as box plots, with the horizontal lines representing the median; the bottom and top of the boxes representing the 25th and 75th percentiles, respectively; and the vertical bars representing the range of the data; any outliers are marked with a circle. Colorectal cancer tissues were compared with matched adjacent normal tissues using the Wilcoxon test (n=336). Representative images of immunohistochemical staining of Smurf1 expression in the same tumour from three cases are shown. Scale bars, 400 μm. (b) Box plot of Smurf1 expression in tumours with different T stages (T Stages 1–4). Any outliers are marked with a circle and extreme cases are marked with an asterisk. Data were analysed using the Kruskal–Wallis test. (c) The percentage of tumours in the four groups of subjects described in (b). Data were analysed using Pearson’sχ2test. (d) Representative images from immunohistochemical staining of Smurf1 expression in two serial sections of the same tumour from four cases in different T stages (T Stages 1–4) are shown. Scale bars, 100 μm. Data were analysed using Pearson’sχ2test. (e) Box plot of Smurf1 expression in tumours with different M stages. Data were analysed using the Mann–WhitneyU-test. (f) The percentage of tumours in the two groups of subjects described in (e). Data were analysed using Pearson’sχ2test. (g) Kaplan–Meier estimates of the cumulative survival rate (n=26). Comparison was made of groups with low Smurf1 expression (scores 0–7), Medium Smurf1 expression (scores 7–8) and high Smurf1 expression (scores 11–12). Marks on graph lines represent censored samples.P-value refers to two-sided log-rank tests. (h) Smurf1-depleted HCT116 cells and control HCT116 cells were injected subcutaneously into the right flank of nude mice. Tumours were isolated after 5 weeks. Figure 1: Smurf1 expression is elevated in colorectal cancer tissues. ( a ) Smurf1 expression scores are shown as box plots, with the horizontal lines representing the median; the bottom and top of the boxes representing the 25th and 75th percentiles, respectively; and the vertical bars representing the range of the data; any outliers are marked with a circle. Colorectal cancer tissues were compared with matched adjacent normal tissues using the Wilcoxon test ( n =336). Representative images of immunohistochemical staining of Smurf1 expression in the same tumour from three cases are shown. Scale bars, 400 μm. ( b ) Box plot of Smurf1 expression in tumours with different T stages (T Stages 1–4). Any outliers are marked with a circle and extreme cases are marked with an asterisk. Data were analysed using the Kruskal–Wallis test. ( c ) The percentage of tumours in the four groups of subjects described in (b). Data were analysed using Pearson’s χ 2 test. ( d ) Representative images from immunohistochemical staining of Smurf1 expression in two serial sections of the same tumour from four cases in different T stages (T Stages 1–4) are shown. Scale bars, 100 μm. Data were analysed using Pearson’s χ 2 test. ( e ) Box plot of Smurf1 expression in tumours with different M stages. Data were analysed using the Mann–Whitney U -test. ( f ) The percentage of tumours in the two groups of subjects described in (e). Data were analysed using Pearson’s χ 2 test. ( g ) Kaplan–Meier estimates of the cumulative survival rate ( n =26). Comparison was made of groups with low Smurf1 expression (scores 0–7), Medium Smurf1 expression (scores 7–8) and high Smurf1 expression (scores 11–12). Marks on graph lines represent censored samples. P -value refers to two-sided log-rank tests. ( h ) Smurf1-depleted HCT116 cells and control HCT116 cells were injected subcutaneously into the right flank of nude mice. Tumours were isolated after 5 weeks. Full size image Nedd8 correlates with Smurf1 expression in colorectal cancer To search for Smurf1 regulators, a yeast two-hybrid screen was performed using the WW-HECT of human Smurf1 as bait, since the WW domains are responsible for substrate recognition, whereas the HECT is the catalytic domain [2] . Twenty preys of potential interacting proteins were obtained ( Supplementary Fig. 2a,b ; Supplementary Table 1 ). One of the recovered interactors, which encodes the full length of Nedd8 protein, attracted our attention for two reasons. First, neddylation has been well defined as an essential activation mechanism of Cullin-RING E3s [4] . The relationship between neddylation and HECT E3s has not been studied. Second, neddylation is functionally related to cancer progression since the specific inhibitor of neddylation E1, MLN4924, is currently being tested in clinical trials for cancer treatment [21] , [22] . MLN4924 disrupts CRL-mediated protein turnover leading to apoptotic death in human tumour cells [21] . We firstly examined the expression of Nedd8 as well as NAE1 (APPBP1), Ubc12 (Nedd8 E2) in colorectal cancer and their possible relationship with Smurf1. An analysis of large-scale subjects (190–283 cases) demonstrated that Nedd8, NAE1 and Ubc12 were all significantly upregulated in colorectal cancer tissues compared with matched adjacent tissues ( Fig. 2a–d ). Importantly, we observed a positive correlation of Smurf1 levels with Nedd8 and NAE1 levels among the examined subjects ( Fig. 2e–g ). By comparison, the correlation between Smurf1 and Ubc12 was not so striking ( Fig. 2h ). To confirm the relevance among Smurf1 and the neddylation enzymatic system, we further examined the expression profile of NEDP1 (also known as DEN1 or SENP8), a cysteine protease specific for Nedd8 (refs 33 , 34 ), and its correlation with Smurf1. We observed that NEDP1 expression was significantly downregulated in cancer tissues compared with adjacent tissues ( Fig. 2i ; Supplementary Fig. 3a ) and it was inversely correlated with Smurf1 levels ( Fig. 2j ; Supplementary Fig. 3b ). 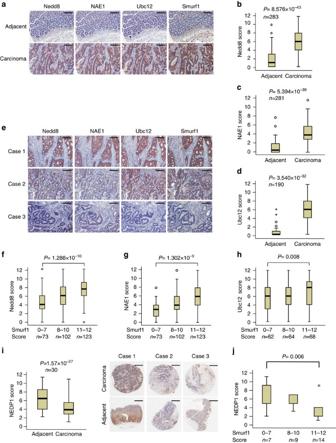Figure 2: Positive correlation of Smurf1 expression with Nedd8 and its interacting enzymes in colorectal cancer. (a) Representative images from immunohistochemical staining of Smurf1, Ubc12, NAE1 and Nedd8 in the same colorectal cancer tumour. Scale bars, 100 μm. (b–d) The expression scores of Nedd8 (b,n=283 ), NAE1 (c,n=281) and Ubc12 (d,n=190) were compared between colorectal cancer tumours and matched adjacent normal tissue using the Wilcoxon test. Any outliers are marked with a circle. (e) Representative images from immunohistochemical staining of Smurf1, Nedd8, NAE1 and Ubc12 expression in four serial sections of the same tumour from three cases. Scale bars, 100 μm. (f–h) Box plot of NAE1, Ubc12 and Nedd8 expression in colorectal cancer from 298 subjects. The subjects were divided into three groups based on Smurf1 expression scores in the tumours, representing low (scores 0–7), medium (scores 8–10) and high (scores 11–12) expression of Smurf1. Data were analysed by Kruskal–Wallis test. (i) Colorectal cancer tissues were compared with matched adjacent normal tissues using the Wilcoxon test (n=30). Any outliers are marked with a circle. Representative images of immunohistochemical staining of NEDP1 expression in the same tumour from three cases are shown. Scale bars, 400 μm. (j) Box plot of NEDP1 expression in colorectal cancer from 30 subjects. The subjects were divided into three groups based on Smurf1 expression scores in the tumours. Data were analysed with the Kruskal–Wallis test. Figure 2: Positive correlation of Smurf1 expression with Nedd8 and its interacting enzymes in colorectal cancer. ( a ) Representative images from immunohistochemical staining of Smurf1, Ubc12, NAE1 and Nedd8 in the same colorectal cancer tumour. Scale bars, 100 μm. ( b – d ) The expression scores of Nedd8 ( b , n =283 ), NAE1 ( c , n =281) and Ubc12 ( d , n =190) were compared between colorectal cancer tumours and matched adjacent normal tissue using the Wilcoxon test. Any outliers are marked with a circle. ( e ) Representative images from immunohistochemical staining of Smurf1, Nedd8, NAE1 and Ubc12 expression in four serial sections of the same tumour from three cases. Scale bars, 100 μm. ( f – h ) Box plot of NAE1, Ubc12 and Nedd8 expression in colorectal cancer from 298 subjects. The subjects were divided into three groups based on Smurf1 expression scores in the tumours, representing low (scores 0–7), medium (scores 8–10) and high (scores 11–12) expression of Smurf1. Data were analysed by Kruskal–Wallis test. ( i ) Colorectal cancer tissues were compared with matched adjacent normal tissues using the Wilcoxon test ( n =30). Any outliers are marked with a circle. Representative images of immunohistochemical staining of NEDP1 expression in the same tumour from three cases are shown. Scale bars, 400 μm. ( j ) Box plot of NEDP1 expression in colorectal cancer from 30 subjects. The subjects were divided into three groups based on Smurf1 expression scores in the tumours. Data were analysed with the Kruskal–Wallis test. Full size image Smurf1 interacts with Nedd8 and Ubc12 We next investigated the interaction of Smurf1 and Nedd8 in HCT116 cells. Endogenous Smurf1 was detected after immunoprecipitation with an anti-Nedd8 antibody ( Supplementary Fig. 4a ). In vitro binding assays indicated direct binding between Smurf1 and Nedd8 ( Supplementary Fig. 4b ). Smurf1 was previously shown to interact with ubiquitin [35] . Consistent with this notion, we confirmed its interaction with ubiquitin, but it was found to be weaker than that with Nedd8 ( Supplementary Fig. 4c ). These interactions were specific because Smurf1 did not interact with SUMO-1, another ubiquitin-like protein ( Supplementary Fig. 4c ). The Smurf1–Nedd8 interaction was dependent on the Ile44-containing hydrophobic surfaceof Nedd8 ( Supplementary Fig. 4d ), a pattern which is similar to the case of ubiquitin–UBD (ubiquitin-binding domain) recognition [36] . Interestingly, Smurf1 contains multiple Nedd8-binding sites. The WW domain, the HECT C-lobe and the HECT N-lobe small subdomain of Smurf1 all possessed the ability to interact with Nedd8 ( Fig. 3d ; Supplementary Fig. 4e ). This is different from the binding region with ubiquitin, since the HECT N-lobe large subdomain specifically interacted with ubiquitin but other domains did not ( Fig. 3d ; Supplementary Fig. 4f ). Consistently, the Smurf1 Y439A mutant, which has been shown to lose the ability to bind to ubiquitin [35] , retained the ability to interact with Nedd8 ( Supplementary Fig. 4g,h ). The HECT N-lobe small subdomain is well defined as the E2 recognition module [2] , implying the possibility that Nedd8 might have an effect on E2 binding to Smurf1. 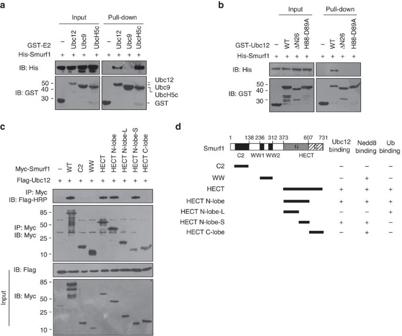Figure 3: Smurf1 interacts with Ubc12. (a) GST pull-down assay of Smurf1 with Ubc12. Both input and pull-down samples were subjected to immunoblotting with anti-His and anti-GST antibodies. Smurf1 interacted with Ubc12 and UbcH5c, but not with Ubc9. (b) Mapping the regions of Ubc12 required for Smurf1 binding. His-Smurf1 and the indicated mutant forms (ΔN26 and H88-D89A) of Ubc12 were used in the GST pull-down assays. (c) Mapping the Ubc12-binding region on Smurf1. Ubc12 and the indicated Smurf1 mutants were transfected into HCT116 cells. Co-immunoprecipitation assays were performed. (d) A schematic diagram of the Ubc12-, Nedd8- and ubiquitin-binding regions of Smurf1 is shown. Figure 3: Smurf1 interacts with Ubc12. ( a ) GST pull-down assay of Smurf1 with Ubc12. Both input and pull-down samples were subjected to immunoblotting with anti-His and anti-GST antibodies. Smurf1 interacted with Ubc12 and UbcH5c, but not with Ubc9. ( b ) Mapping the regions of Ubc12 required for Smurf1 binding. His-Smurf1 and the indicated mutant forms (ΔN26 and H88-D89A) of Ubc12 were used in the GST pull-down assays. ( c ) Mapping the Ubc12-binding region on Smurf1. Ubc12 and the indicated Smurf1 mutants were transfected into HCT116 cells. Co-immunoprecipitation assays were performed. ( d ) A schematic diagram of the Ubc12-, Nedd8- and ubiquitin-binding regions of Smurf1 is shown. Full size image Given that Smurf1 is a typical E3 ligase, we next examined whether Smurf1 can bind the Nedd8 E2, Ubc12. In vitro binding assays revealed that Smurf1 could bind to Ubc12 and to the ubiquitin E2, UbcH5c, but not the SUMO E2, Ubc9 ( Fig. 3a ). This binding was unaffected by the Smurf1 C699A mutation ( Supplementary Fig. 4i ), which abolishes its ubiquitin ligase activity [30] . The binding of E3 ligases to E2s often occurs on the surface of the E2 that is recognized by its corresponding E1 enzyme [37] . The E1 interaction site of Ubc12 requires the H88 and D89 residues within the αβ core domain and amino acids 1–26 within the N-terminal region [38] . Strikingly, Smurf1 could no longer bind to Ubc12 if the Ubc12 H88A-D89A or ΔN26 mutant was tested for interaction ( Fig. 3b ). Thus, the Ubc12 sites for binding to Smurf1 appear to largely overlap with that for the E1. The previously identified Nedd8 ligation-promoting factor Dcn1 binds Ubc12 in the same pattern [23] . In addition, deletion analysis indicated that the Smurf1 HECT N-lobe small subdomain mediated the interaction with Ubc12 ( Fig. 3c,d ). This subdomain also mediates the interaction with the ubiquitin E2 (ref. 2 ). Thus, Smurf1 interacts with Ubc12 in a typical E3–E2 recognition pattern, suggesting that Smurf1 might function as a Nedd8 ligase. Smurf1 catalyses its own neddylation through C426 active site We next investigated whether Smurf1 can be conjugated with Nedd8. We first performed in vitro neddylation assays with purified Smurf1, Nedd8, NAE (E1), Ubc12 (E2). The results showed that Smurf1 migrated as high-molecular weight bands when the Nedd8, NAE and Ubc12 are present in the reaction ( Fig. 4a ). These conjugations were independent of the ubiquitin ligase activity of Smurf1, since the ubiquitin ligase catalytic-inactive mutant C699A was conjugated similar to Smurf1 WT ( Fig. 4a ). To verify these conjugations are neddylations, we incubated the components with the Nedd8-specific protease NEDP1. We found that NEDP1 WT removed these conjugation bands but the NEDP1 catalytic-inactive C163A mutant did not ( Fig. 4b ), suggesting that these conjugations are neddylations. We next investigated whether Smurf1 is neddylated in vivo . Immunoprecipitation of the HCT116 cell lysates with an Nedd8-specific antibody showed that endogenous Smurf1 was detectable as smear bands in the immunoprecipitates ( Fig. 4c ; Fig. 5b ). These immunoprecipitated proteins were not recognized by the ubiquitin antibody, and vice versa ( Fig. 4c ). These smear bands of Smurf1 were eliminated by treatment with MLN4924 ( Fig. 4d ), a potent and specific inhibitor of the NAE. Depletion of Uba3, the NAE1 subunit of Nedd8 E1 heterodimer, or depletion of Ubc12, the Nedd8 E2, resulted in a dramatic reduction of the smear bands ( Fig. 4e ). In addition, these smear bands disappeared if a Nedd8-ΔGG mutant, which abolishes the covalent conjugating ability of Nedd8, was used in the neddylation assays ( Fig. 4f , lane 4), suggesting that these bands represent neddylated Smurf1 proteins. Collectively, Smurf1 was neddylated both in vitro and in the cultured cells, and the modification was not due to the mixture of Nedd8 and ubiquitin. 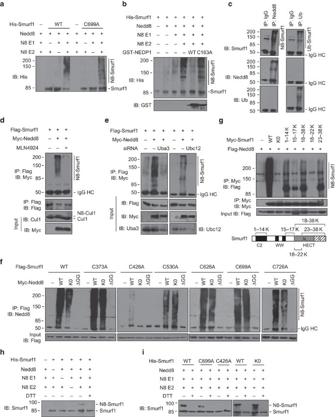Figure 4: Nedd8 is attached to Smurf1 through C426-catalysed autoneddylation. (a) Covalent neddylation of Smurf1in vitro.Purified His-Smurf1-WT or C699A proteins were incubated with Nedd8 and Nedd8-E1/E2. Reactions were performed as described in the Methods section. Samples were analysed by western blotting with an anti-His antibody. (b) Deneddylation enzyme NEDP1 abolished covalent neddylation of Smurf1in vitro.Neddylated Smurf1 was purified on Ni2+-NTA Superflow Cartridges (QIAGEN) and then incubated with GST-NEDP1 WT or C163A. Reactions were performed as described in the Methods. Samples were analysed by western blotting with an anti-His antibody. (c)In vivoneddylation and ubiquitylation assay were used to detect covalent modification of endogenous Smurf1. HCT116 cells (1 × 109) were solubilized in modified lysis buffer and immunoprecipitated with the Nedd8 and ubiquitin antibodies. (d,e) Smurf1 was neddylated in mammalian cells. Smurf1 neddylation was significantly attenuated by the NAE inhibitor MLN4924 or depletion of Uba3 (one subunit of NAE) or Ubc12. The indicated plasmids or siRNAs were transfected into HCT116 cells. Flag antibody-immunoprecipitated Smurf1 proteins were analysed by immunoblotting with an anti-Myc antibody to detect conjugated Nedd8. (f) Smurf1-WT and the indicated CA mutants were co-transfected with Nedd8 WT, K0 or ΔGG to detect covalently modified Smurf1 in HCT116 cells. (g)In vivoSmurf1 neddylation assay. HEK293T cells were transfected with Flag-Nedd8, Myc-tagged Smurf1 WT and mutants, including K0 (all 38 Lys residues mutated to Arg), 1–14 K (only retained lysines in the C2 domain), 15–17 K (in the WW-HECT linker), 18–38 K (in the HECT domain), 18–22 K (in the N-terminal region of HECT), 23–38 K (in the resting region of HECT). The cells were harvested and subjected to neddylation asssy 48 h after transfection. A schematic diagram of the lysine sites on Smurf1 is shown. * means none-specific band. (h,i)In vitroNedd8-thioester bond assays. Smurf1 WT and K0 mutants were expressed in bacteria and purified. Figure 4: Nedd8 is attached to Smurf1 through C426-catalysed autoneddylation. ( a ) Covalent neddylation of Smurf1 in vitro. Purified His-Smurf1-WT or C699A proteins were incubated with Nedd8 and Nedd8-E1/E2. Reactions were performed as described in the Methods section. Samples were analysed by western blotting with an anti-His antibody. ( b ) Deneddylation enzyme NEDP1 abolished covalent neddylation of Smurf1 in vitro. Neddylated Smurf1 was purified on Ni 2+ -NTA Superflow Cartridges (QIAGEN) and then incubated with GST-NEDP1 WT or C163A. Reactions were performed as described in the Methods. Samples were analysed by western blotting with an anti-His antibody. ( c ) In vivo neddylation and ubiquitylation assay were used to detect covalent modification of endogenous Smurf1. HCT116 cells (1 × 10 9 ) were solubilized in modified lysis buffer and immunoprecipitated with the Nedd8 and ubiquitin antibodies. ( d , e ) Smurf1 was neddylated in mammalian cells. Smurf1 neddylation was significantly attenuated by the NAE inhibitor MLN4924 or depletion of Uba3 (one subunit of NAE) or Ubc12. The indicated plasmids or siRNAs were transfected into HCT116 cells. Flag antibody-immunoprecipitated Smurf1 proteins were analysed by immunoblotting with an anti-Myc antibody to detect conjugated Nedd8. ( f ) Smurf1-WT and the indicated CA mutants were co-transfected with Nedd8 WT, K0 or ΔGG to detect covalently modified Smurf1 in HCT116 cells. ( g ) In vivo Smurf1 neddylation assay. HEK293T cells were transfected with Flag-Nedd8, Myc-tagged Smurf1 WT and mutants, including K0 (all 38 Lys residues mutated to Arg), 1–14 K (only retained lysines in the C2 domain), 15–17 K (in the WW-HECT linker), 18–38 K (in the HECT domain), 18–22 K (in the N-terminal region of HECT), 23–38 K (in the resting region of HECT). The cells were harvested and subjected to neddylation asssy 48 h after transfection. A schematic diagram of the lysine sites on Smurf1 is shown. * means none-specific band. ( h , i ) In vitro Nedd8-thioester bond assays. Smurf1 WT and K0 mutants were expressed in bacteria and purified. 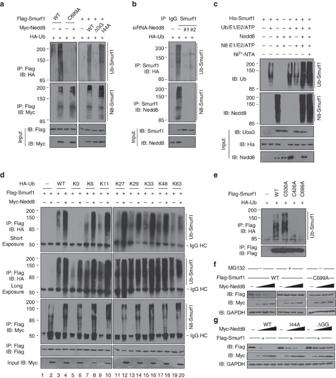Figure 5: Neddylation of Smurf1 activates its ubiquitin ligase activity. (a)In vivoSmurf1 ubiquitylation assay. Nedd8 was co-expressed with Smurf1 WT or C699A in HCT116 cells (left panels). Twenty-four hours post transfection, cells were treated with MG132 (20 μM, 8 h). HCT116 cells were transfected with a constant amount of Smurf1 with Nedd8 WT, I44A or ΔGG, and Smurf1 ubiquitylation (right panels). Cells were treated with MG132 (20 μM, 8 h) before being harvested. (b)In vivoSmurf1 ubiquitylation assay with Nedd8 depletion. Cells were treated with MG132 (20 μM) for 8 h. (c)In vitroSmurf1 ubiquitylation assay in the presence of Nedd8-E1/E2, Nedd8 WT or ΔGG. Neddylated Smurf1 was purified on Ni2+-NTA Superflow Cartridges and then incubated with ubquitin E1 and E2(UbcH5c). (d)In vivoSmurf1 ubiquitylation assay. HEK293T cells were transfected with Flag-Smurf1, Myc-Nedd8 and different HA-tagged ubiquitin mutants. The K0 denotes ubiquitin mutant with all 7 Lys residues mutated to Arg, and K6, K11, K27, K29, K33, K48 or K63 are mutants of ubiquitin that only have the indicated Lys residue. The cells were treated with MG132 before being harvested and subjected to ubiquitylation asssy 48 h after transfection. (e)In vivoubiquitylation assay for Smurf1 WT and the indicated CA mutants in HCT116 cells. MG132 was added into the cells before being harvested. (f) Nedd8 was co-expressed with Smurf1 WT or C699A in HCT116 cells. Twenty-four hours post transfection, cells were treated with MG132 (20 μM, 8 h). (g) HCT116 cells were transfected with a constant amount of Smurf1 with Nedd8 WT, I44A or ΔGG, and Smurf1 protein levels were determined. Full size image Figure 5: Neddylation of Smurf1 activates its ubiquitin ligase activity. ( a ) In vivo Smurf1 ubiquitylation assay. Nedd8 was co-expressed with Smurf1 WT or C699A in HCT116 cells (left panels). Twenty-four hours post transfection, cells were treated with MG132 (20 μM, 8 h). HCT116 cells were transfected with a constant amount of Smurf1 with Nedd8 WT, I44A or ΔGG, and Smurf1 ubiquitylation (right panels). Cells were treated with MG132 (20 μM, 8 h) before being harvested. ( b ) In vivo Smurf1 ubiquitylation assay with Nedd8 depletion. Cells were treated with MG132 (20 μM) for 8 h. ( c ) In vitro Smurf1 ubiquitylation assay in the presence of Nedd8-E1/E2, Nedd8 WT or ΔGG. Neddylated Smurf1 was purified on Ni 2+ -NTA Superflow Cartridges and then incubated with ubquitin E1 and E2(UbcH5c). ( d ) In vivo Smurf1 ubiquitylation assay. HEK293T cells were transfected with Flag-Smurf1, Myc-Nedd8 and different HA-tagged ubiquitin mutants. The K0 denotes ubiquitin mutant with all 7 Lys residues mutated to Arg, and K6, K11, K27, K29, K33, K48 or K63 are mutants of ubiquitin that only have the indicated Lys residue. The cells were treated with MG132 before being harvested and subjected to ubiquitylation asssy 48 h after transfection. ( e ) In vivo ubiquitylation assay for Smurf1 WT and the indicated CA mutants in HCT116 cells. MG132 was added into the cells before being harvested. ( f ) Nedd8 was co-expressed with Smurf1 WT or C699A in HCT116 cells. Twenty-four hours post transfection, cells were treated with MG132 (20 μM, 8 h). ( g ) HCT116 cells were transfected with a constant amount of Smurf1 with Nedd8 WT, I44A or ΔGG, and Smurf1 protein levels were determined. Full size image Smurf1 can be neddylated by itself or by other Nedd8 ligase(s). Among the currently known Nedd8 ligases (that is, Dcn1, Roc1/Rbx1, MDM2, IAPs and c-Cbl) [6] , [13] , [23] , [25] , [39] , [40] , [41] , [42] , only MDM2 was demonstrated to interact with Smurf1 (ref. 43 ). MDM2 promotes the neddylation of p53 as well as itself [6] . However, under our experimental conditions, MDM2 overexpression did not enhance Smurf1 neddylation. As a positive control, neddylation of p53 was significantly enhanced by MDM2 ( Supplementary Fig. 5a ). Smurf1 was still neddylated even in MDM2-deficient MEF cells ( Supplementary Fig. 5b ), suggesting that MDM2 was not required for Smurf1 neddylation. We noted that most of the currently known Nedd8 ligases also function as ubiquitin ligases. The facts that Smurf1 was effectively neddylated in the absence of any other Nedd8 E3 under the in vitro conditions ( Fig. 4a ) and that Smurf1 interacts with Nedd8 and Ubc12 ( Fig. 3 ) prompted us to hypothesize that Smurf1 can function as a Nedd8 ligase to catalyse its own neddylation. If this is true, which cysteine functions as the catalytic acitive site? The result in Fig. 4a excluded C699 as the active site. To identify the active cysteine, each cysteine in the Smurf1 HECT domain was mutated into alanine, and neddylation assays were performed. This revealed C426, which is located in the HECT N-lobe, as the responsible active site ( Fig. 4f ; Supplementary Fig. 6a ). Smurf1 C426 is conserved across species ( Supplementary Fig. 6b ). Mutation of C426A resulted in a decrease in Smurf1 autoneddylation to a level similar to that of Smurf1 in the presence of MLN4924 treatment or Uba3 and Ubc12 depletion ( Supplementary Fig. 6c–e ). Smurf1 catalyses mono-neddylation on multiple lysines We next attempted to identify the neddylation sites in Smurf1. We noted that Smurf1 neddylation by Nedd8-K0 (lysine zero), in which all lysines in Nedd8 were mutated to arginines to prevent Nedd8 chain formation, was not significantly reduced compared with neddylation by Nedd8 WT ( Fig. 4f ), suggesting that Smurf1 might be predominantly mono-neddylated at multiple lysines. Mass-spectrometry (MS) analysis was performed to determine which lysines are modified. Given that full-length Smurf1 easily degrades in vitro under our conditions with unknown mechanism, we attempted to identify the modified lysines using the Smurf1 mutant consisting of WW plus HECT domains, which was relatively stable compared with the full-length protein. We identified six lysine sites of Smurf1 that were auto-neddylated in vitro : K324, K495, K545, K558, K559 and K667 ( Supplementary Fig. 7a,b ). Among these sites, K324 is located within the linker between WW and HECT domains, whereas the other five sites are within the HECT domain. However, mutation of all of these lysines to arginines did not abolish the neddylation of Smurf1 ( Supplementary Fig. 7b ), suggesting that other unidentified sites exist in the WW-HECT region. Scanning of Smurf1 sequence showed that it contains a total of 38 lysines, including 14 lysines in the C2 domain, 3 lysines in the WW-HECT linker and 21 lysines in the HECT domain. We mutated all of the 38 lysines to arginines to generate a K0 mutant, and confirmed that it indeed could not be neddylated ( Fig. 4g ). Based on this K0 mutant, we then constructed a series of mutants in which the lysines were restored according to the Smurf1 domains. This strategy generated 1–14 K (this mutant contains the first 14 lysines located in the C2 domain), 15–17 K (in WW-HECT linker), 18–38 K (in the HECT domain), and two more mutants, that is, 18–22 K (a cluster in the N-terminal region of HECT) and 23–38 K (in the resting region of HECT). Figure 4g of in vivo neddylation assays clearly showed that (1) Smurf1 18–22 K could not be neddylated, indicating that these five lysines were not neddylation sites; (2) Smurf1 15–17 K was mono-neddylated, which is consistent with the MS data that K324 (it is the 15th lysine) was neddylated; (3) Smurf1 1–14 K and 23–38 K were multi-neddylated and the neddylation of each mutant was reduced compared with the Smurf1 WT, suggesting that multiple neddylation sites were located in the C2 domain and the C-terminal part of HECT domain. Consistent with this hypothesis, K495, K545, K558, K559 and K667, which were identified by MS, are all located in the C-terminal part of HECT domain (23–38 K). These findings indicate that Smurf1 was neddylated on multiple lysine sites in the C2, HECT domains and the WW-HECT linker region, which is different from the mono-neddylation of Cullins. Smurf1 C426 forms a thioester bond with Nedd8 To test whether Smurf1 can form an obligate thioester bond with Nedd8, a thioester bond formation assay was performed. A DTT-sensitive mono-Nedd8 thioester adduct was detected ( Fig. 4h ). The C426A mutation prevented the formation of the thioester intermediate ( Fig. 4i ). In comparison, C699A mutation had no effect on the Smurf1-Nedd8 thioester bond formation ( Fig. 4i ). Smurf1 K0 mutant also formed this Nedd8-thioester bond ( Fig. 4i ), confirming that the band was not an isopeptide bond that should be formed with a lysine residue. Neddylation of Smurf1 promotes its ubiquitin ligase activity To determine the possible regulatory role of neddylation on Smurf1 ubiquitin ligase activity, we first investigated the effects of Nedd8 on Smurf1 autoubiquitylation in vivo . Ectopic expression of Nedd8 increased the autoubiquitylation of wild-type Smurf1, but not its ligase-defective C699A mutant ( Fig. 5a ). This effect was dependent on the diglycine (GG) motif-mediated covalent conjugation ( Fig. 5a ). Conversely, depletion of Nedd8 by two independent siRNAs attenuated Smurf1 autoubiquitylation ( Fig. 5b ). Depletion of Ubc12 also resulted in decreased Smurf1 autoubiquitylation ( Supplementary Fig. 8a ). Next we examined the effects of neddylation on Smurf1 ubiquitylation in vitro . We reconstituted the ubiquitylation of Smurf1 in vitro using purified ubiquitin E1, E2 (UbcH5c), Smurf1, in the absence or presence of Nedd8, Nedd8 E1 and E2 (Ubc12). In this system, Nedd8 or Nedd8 E1/E2 alone did not substantially augment the autoubiquitylation of Smurf1 ( Fig. 5c , lanes 5 and 6 versus lane 2). When Nedd8, Nedd8 E1 and E2 were all included, the autoubiquitylation of Smurf1 was significantly enhanced (lane 7), suggesting that Nedd8 augmented Smurf1 activity in vitro also in a covalent conjugation-dependent manner. To confirm that the enhancing effects were attributed to the neddylated Smurf1, we purified the neddylated Smurf1 using Ni 2+ -NTA Superflow before the in vitro ubiquitylation reaction. To prove these proteins were purified Smurf1 but did not contain other components, we analysed Nedd8 E1 and Nedd8 with western blot. The results showed that Nedd8 E1 and Nedd8 were undetectable in the purified proteins ( Fig. 5c , lane 8). Ubiquitylation assays showed that the purified neddylated Smurf1 effectively promoted the Smurf1 autoubiquitylation (lane 8). Furthermore, we compared two ubiquitin E2s, UbcH5c and UbcH7, in the assays. We obtained similar results that Nedd8 promoted the ubiquitin transfer from E2 to Smurf1 ( Supplementary Fig. 8b,c ). Therefore, neddylation promotes Smurf1 activity both in vivo and in vitro . We next investigated the types of ubiquitin chains of Smurf1 that were affected by neddylation. We used a panel of ubiquitin mutants in which all lysines were mutated into arginines (K0, which can only mono-ubiquitylate protein) or only one lysine (K6, K11, K27, K29, K33, K48 or K63) was retained. As shown in Fig. 5d , Smurf1 could be conjugated to all types of polyubiquitin linkage (lanes 7, 9, 11, 13, 15, 17 and 19). Smurf1 could be also mono-ubiquitylated (lane 5); however, this seemed weaker than the polyubiquitylation. Ectopic expression of Nedd8 enhanced most types of polyubiquitin linkage of Smurf1 significantly (lanes 8, 10, 12, 14, 16 and 18) and also the mono-ubiquitylation (lane 6), except for the weak effect on K63 linkage (lane 20). These results suggested that Nedd8 primarily promoted the degradative polyubiquitylation of Smurf1. The critical role of neddylation on Smurf1 ligase activation was confirmed by the result that Smurf1 C426A mutant, like C699A, almost completely lost the ability to catalyse autoubiquitylation ( Fig. 5e ). Analysis of Smurf1 steady-state levels showed that ectopic expression Nedd8 enhanced the Smurf1 turnover by autoubiquitylation and proteasomal degradation ( Fig. 5f ) but had no effects on Smurf1 mRNA levels ( Supplementary Fig. 8d ). This regulation was also dependent on covalent conjugation ( Fig. 5g ). Overexpression of a dominant-negative mutant of Ubc12 resulted in increased Smurf1 levels ( Supplementary Fig. 8e ). Co-expression of deneddylase NEDP1, but not with its inactive mutant, eliminated the effects of Nedd8 on Smurf1 ( Supplementary Fig. 8f ). Collectively, these results indicate that Nedd8 augments the ligase activity of Smurf1 via covalent conjugation. Neddylation enhances Smurf1-mediated ubiquitination We sought to test whether Nedd8 could enhance the activity of Smurf1 towards its substrates, including Smad4, Smad5, RhoA and ING2 (refs 27 , 44 , 45 , 46 ). For Smad4 degradation, Smurf1 needs the adaptor role of Smad7 since Smurf1 cannot bind to Smad4 directly [45] . Co-expression of Nedd8 with Smurf1 and Smad7 markedly decreased Smad4 levels and promoted Smad4 ubiquitylation in a covalent conjugation-dependent manner ( Fig. 6a,b ). Likewise, Nedd8 promoted the ability of Smurf1 to ubiquitylate and degrade Smad5, RhoA or ING2 ( Supplementary Fig. 9a–c ). 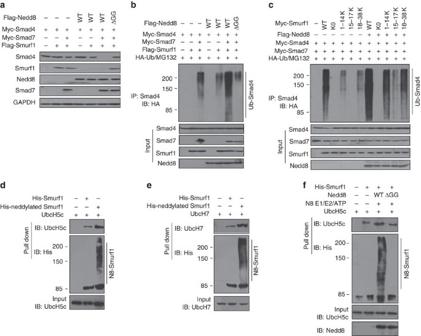Figure 6: Neddylation of Smurf1 enhances E2 binding and promotes the substrate ubiquitylation. (a) Smad4, Smad7, Smurf1 and Nedd8 were co-transfected into HCT116 cells. Cell lysates were immunoblotted to detect Smad4 levels. (b,c)In vivoubiquitylation assay of Smad4. The indicated Nedd8 mutants (b) or Smurf1 mutants (c) were co-transfected with Smad4, Smurf1 and ubiquitin into HCT116 cells. Twenty-four hours post-transfection, cells were treated with MG132 (20 μM, 8 h). (d,e) Neddylation enhances ubiquitin E2 binding to Smurf1. Bacterially expressed Ub E2 (UbcH5c or UbcH7) were incubated within vitroneddylated Smurf1 or unneddylated Smurf1 proteins. Both input and pull-down samples were subjected to immunoblotting with the indicated antibodies. (f) Nedd8 WT or ΔGG mutant was incubated with UbcH5c, Smurf1 and the neddylation E1/E2. Interaction between Smurf1 and UbcH5c was measured. Figure 6: Neddylation of Smurf1 enhances E2 binding and promotes the substrate ubiquitylation. ( a ) Smad4, Smad7, Smurf1 and Nedd8 were co-transfected into HCT116 cells. Cell lysates were immunoblotted to detect Smad4 levels. ( b , c ) In vivo ubiquitylation assay of Smad4. The indicated Nedd8 mutants ( b ) or Smurf1 mutants ( c ) were co-transfected with Smad4, Smurf1 and ubiquitin into HCT116 cells. Twenty-four hours post-transfection, cells were treated with MG132 (20 μM, 8 h). ( d , e ) Neddylation enhances ubiquitin E2 binding to Smurf1. Bacterially expressed Ub E2 (UbcH5c or UbcH7) were incubated with in vitro neddylated Smurf1 or unneddylated Smurf1 proteins. Both input and pull-down samples were subjected to immunoblotting with the indicated antibodies. ( f ) Nedd8 WT or ΔGG mutant was incubated with UbcH5c, Smurf1 and the neddylation E1/E2. Interaction between Smurf1 and UbcH5c was measured. Full size image We then examined the effects of Smurf1 mutants on substrate (Smad4) ubiquitylation. The Smad4 ubiquitylation, both in the absence and presence of ectopic Nedd8,was dramatically enhanced by wild-type Smurf1, moderately enhanced by Smurf1 1–14 K and 18–38 K, and weakly enhanced by Smurf1 15–17 K; in contrast, it was hardly detectable in the case of Smurf1 K0 ( Fig. 6c ). The data suggest that multiple-site neddylation of Smurf1 was required for Smurf1 to efficiently ubiquitylate Smad4. Some of the monitored Smurf1 substrates are also substrates of CRLs. For example, Smad4 is ubiquitylated by SCF β-TrCP target [47] , while RhoA is targeted by CRL3 (ref. 48 ). To confirm that the effects of Nedd8 on these substrates are through Smurf1, at least partially, we knocked down endogenous Roc1/Rbx1, one essential component of CRL (ref. 1 ), by RNAi. Under these conditions, ectopic expression of Smurf1 still had significant enhancing effects on the ubiquitylation of Smad5 and RhoA, and promoted their degradation ( Supplementary Fig. 9d–f ). In addition, although Roc1 was knocked down, co-expression of Nedd8 with Smurf1 still significantly decreased Smad4 levels and promoted its ubiquitylation, whose effects were dependent on C426-mediated Smurf1 autoneddylation ( Supplementary Fig. 9g–i ). Therefore, these data suggest that Nedd8 can regulate Smad4, Smad5 and RhoA protein levels and ubiquitylation through activation of Smurf1, which provides an alternative regulatory mechanism besides the CRLs. Neddylation enhances ubiquitin E2 binding to Smurf1 Neddylation promotes E2 recruitment in Cullins [49] , [50] . We investigated whether neddylation had any effects on Smurf1 interaction with ubiquitin E2. The binding of purified UbcH5c or UbcH7 proteins to purified in vitro neddylated Smurf1or unneddylated Smurf1 was examined. The results showed that Smurf1 alone could bind to UbcH5c and UbcH7. Neddylated Smurf1 bound more UbcH5c or UbcH7 than unneddylated Smurf1 ( Fig. 6d,e ) and the enhanced binding ability was dependent on the GG motif of Nedd8, which was required for covalent conjugation ( Fig. 6f ). In addition, Nedd8 had no significant effects on the interactions of Smurf1 with its substrates ( Supplementary Fig. 9j ). These results indicate that neddylation enhanced the interaction between E2 and Smurf1, which may explain why covalent conjugation of Nedd8 promotes Smurf1 activity. Therefore, similar to the behaviour of Nedd8 on Cullins, the rule that neddylation enhances E2–E3 interaction is also utilized by HECT-type E3s. Neddylation is also critical for E3 activity of yeast Rsp5 Smurf1 belongs to the Nedd4 family of C2-WW-HECT E3s, which are evolutionarily conserved through yeast to mammals [51] , [52] . To extend our findings, we investigated whether neddylation plays a role in the activation of Rsp5 ( Fig. 7a ), the single Smurf1 homologue that exists in Saccharomyces cerevisiae . Rub1, the yeast homologue of Nedd8, formed conjugates at the molecular weight similar to Rsp5; the conjugation was dependent on E1 (that is, Uba3 and Ula1) and E2 (Ubc12) ( Supplementary Fig. 10a ). Human Nedd8 could also form conjugates in yeast ( Supplementary Fig. 10b ). Rsp5 formed upshifted bands when co-expressed with Rub1 but not with the GG-deleted version of Rub1 ( Fig. 7b,c ). C777 is the active cysteine for Rsp5 ubiquitin ligase activity. We demonstrated that a C777A mutation in Rsp5 abolished its Rub1 conjugation ( Fig. 7d ), suggesting that Rsp5 uses a single active site for ubiquitin and Nedd8 ligation. In addition, the modification of Rsp5 by Rub1 was dependent on E1 and E2 ( Fig. 7e ). Furthermore, the diglycine residue-conjugated sites were identified by LC-MS/MS analysis ( Supplementary Fig. 10c,d and Supplementary Data 1 and 2 ). Combined with data from the substitution mutants, we identified K45 as the autoneddylation site of Rsp5 ( Fig. 7f ). 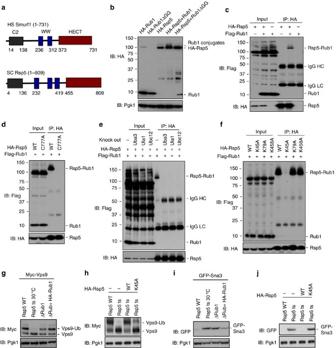Figure 7: Yeast Rsp5 ubiquitin ligase is also activated by neddylation. (a) Schematic diagram of human Smurf1 and yeast Rsp5. (b) Rsp5 could form upshifted bands when co-expressed with Rub1. Rsp5 expression plasmids were transformed into yeast Rub1-knockout cells alone or together with wild-type Rub1 or the GG-deleted version of Rub1. Cells were collected and lysed for western blot. Upshifted bands were detected when Rsp5 was co-expressed with wild-type Rub1 but not with the GG-deleted version of Rub1. (c)Yeast cells expressing HA-Rsp5, Flag-Rub1 or both were subjected to immunoprecipitation with HA antibody beads. Western blots were performed to detect Rub1-modified Rsp5. (d) Mutation of the C777 active site of Rsp5 abolishes its Rub1 conjugation. (e) The modification of Rsp5 by Rub1 is dependent on the Rub1 conjugation pathway E1 and E2. Rsp5 and Rub1 were co-transfected into wild-type or Uba3-, Ula1-, Ubs12-knockout yeast cells. Immunoprecipitation and western blot were performed to detect Rub1 modification of Rsp5. (f) Mutation of K45A in Rsp5 abolishes the Rub1 modification. Wild-type or lysine to alanine mutants of Rsp5 were co-expressed with Rub1 in yeast cells. Rub1 conjugation to Rsp5 was detected by immunoprecipitation and subsequent western blot. (g,h) Rub1 modification of Rsp5 is important for the ubiquitylation of its substrate Vps9. Vps9 was chromosomally tagged with a myc tag in different yeast cells, as indicated. The upshifted band of Vps9 demonstrates its ubiquitylation. (i,j) Rub1 modification of Rsp5 is important for its function in the degradation of membrane protein Sna3. Sna3 was chromosomally tagged with a GFP tag in different yeast cells, and its protein levels were detected by western blot. Figure 7: Yeast Rsp5 ubiquitin ligase is also activated by neddylation. ( a ) Schematic diagram of human Smurf1 and yeast Rsp5. ( b ) Rsp5 could form upshifted bands when co-expressed with Rub1. Rsp5 expression plasmids were transformed into yeast Rub1-knockout cells alone or together with wild-type Rub1 or the GG-deleted version of Rub1. Cells were collected and lysed for western blot. Upshifted bands were detected when Rsp5 was co-expressed with wild-type Rub1 but not with the GG-deleted version of Rub1. ( c )Yeast cells expressing HA-Rsp5, Flag-Rub1 or both were subjected to immunoprecipitation with HA antibody beads. Western blots were performed to detect Rub1-modified Rsp5. ( d ) Mutation of the C777 active site of Rsp5 abolishes its Rub1 conjugation. ( e ) The modification of Rsp5 by Rub1 is dependent on the Rub1 conjugation pathway E1 and E2. Rsp5 and Rub1 were co-transfected into wild-type or Uba3-, Ula1-, Ubs12-knockout yeast cells. Immunoprecipitation and western blot were performed to detect Rub1 modification of Rsp5. ( f ) Mutation of K45A in Rsp5 abolishes the Rub1 modification. Wild-type or lysine to alanine mutants of Rsp5 were co-expressed with Rub1 in yeast cells. Rub1 conjugation to Rsp5 was detected by immunoprecipitation and subsequent western blot. ( g , h ) Rub1 modification of Rsp5 is important for the ubiquitylation of its substrate Vps9. Vps9 was chromosomally tagged with a myc tag in different yeast cells, as indicated. The upshifted band of Vps9 demonstrates its ubiquitylation. ( i , j ) Rub1 modification of Rsp5 is important for its function in the degradation of membrane protein Sna3. Sna3 was chromosomally tagged with a GFP tag in different yeast cells, and its protein levels were detected by western blot. Full size image Next, we assayed whether Rub1-mediated modification of Rsp5 would affect its ligase activity during endocytosis. Vps9, a guanine nucleotide exchange factor required for efficient endocytosis, is a well-characterized mono-ubiquitylation substrate of Rsp5 (ref. 53 ). We examined ubiquitylation of Vps9 in a yeast strain that carried a temperature-conditional allele of Rsp5 (Rsp5-ts). Western blot analysis of cell extracts generated from the Rsp5-WT and Rsp5-ts yeast strains at a nonpermissive temperature (30 °C) revealed the presence of ubiquityl-Vps9 in only the wild-type strain ( Fig. 7g ).When this strain lacked Rub1, the level of ubiquitylated Vps9 was markedly reduced. The decrease of ubiquitylated Vps9 in Rub1-deleted strain was partially rescued by ectopic Rub1 ( Fig. 7g ). Next we transformed wide type or K45A mutant of Rsp5 back into Rsp5-ts cells, and checked the ubiquitination of Vps9. The results showed that without Rub1 modification of Rsp5 on K45, the ubiquitination of Vps9 by Rsp5 was decreased ( Fig. 7h ; Supplementary Fig. 10e ). These findings demonstratethat Rub1-mediated modification of Rsp5 is important for the ubiquitylation of Vps9. In addition, Rsp5 promotes the polyubiquitylation and degradation of membrane proteins, such as the multivesicular bodies cargo Sna3 (refs 54 , 55 ). We showed that Rub1 modification of Rsp5 on K45 was important for the degradation of Sna3 by Rsp5 ( Fig. 7i,j ). Thus, Rub1 modification significantly upregulates Rsp5 function in yeast cells. Nedd8-mediated Smurf1 activation promotes cancer progression The above results suggest that Smurf1 is not only highly expressed in colorectal cancer tissues but also activated by co-expressed Nedd8, NAE and Ubc12. To gain insight into the role of Smurf1 autoneddylation in cancer progression, we examined the effects of Smurf1 C426A on tumour growth in both cultured cells and nude mice. We reintroduced shRNA-resistant Smurf1-WT, C426A, C530A or C699A into Smurf1-depleted HCT116 cells ( Fig. 8a ). Reintroduction of Smurf1-WT or C530A significantly augmented tumour weight and volume in nude mice ( Fig. 8b–d ) and promoted cell proliferation and tumour invasion in cultured cells ( Fig. 8e,f ). In contrast, the reintroduction of Smurf1 C426A or C699A into these cells caused a weak or insignificant increase in tumour growth and invasion ( Fig. 8b–f ). These data demonstrate that the autoneddylation-mediated activation of Smurf1 is required for its tumour-promoting effects. 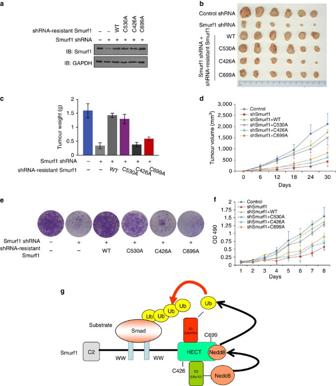Figure 8: Neddylation-mediated Smurf1 activation promotes the progression of colorectal cancer. (a) Smurf1 WT or C426A, C530A, C699A mutant vectors were each stably transfected into HCT116 cells that were depleted of Smurf1 using a Lentivirus-coupled shRNA against Smurf1. The expression of Smurf1 was detected by western blot to determine the efficiency of depletion (lane 2) and to compare expression levels among the overexpression groups (lanes 3–6). (b) Volume of xenograft tumours derived from HCT116 cells (5 × 106per mouse) subcutaneously inoculated into the right flank of the mice (n=6 in each group). The transplanted tumours were removed and photographed. (c) Six nude mice were injected subcutaneously for each of the indicated stable cell lines. Tumours were isolated, and their weights were measured. (d) TV was measured using a caliper at the indicated time points. Data are shown as the mean±s.d. (e) Thein vitrocell migration assay was performed in transwell plates. Representative results from three independent experiments are shown. (f) An MTS assay was performed. Cell proliferation was assessed every 24 h. Data are presented as the mean±s.d. Results are from a representative experiment performed in triplicate. (g) Working model of Nedd8-mediated conjugation on the activation of Smurf1 ubiquitin ligase. Figure 8: Neddylation-mediated Smurf1 activation promotes the progression of colorectal cancer. ( a ) Smurf1 WT or C426A, C530A, C699A mutant vectors were each stably transfected into HCT116 cells that were depleted of Smurf1 using a Lentivirus-coupled shRNA against Smurf1. The expression of Smurf1 was detected by western blot to determine the efficiency of depletion (lane 2) and to compare expression levels among the overexpression groups (lanes 3–6). ( b ) Volume of xenograft tumours derived from HCT116 cells (5 × 10 6 per mouse) subcutaneously inoculated into the right flank of the mice ( n =6 in each group). The transplanted tumours were removed and photographed. ( c ) Six nude mice were injected subcutaneously for each of the indicated stable cell lines. Tumours were isolated, and their weights were measured. ( d ) TV was measured using a caliper at the indicated time points. Data are shown as the mean±s.d. ( e ) The in vitro cell migration assay was performed in transwell plates. Representative results from three independent experiments are shown. ( f ) An MTS assay was performed. Cell proliferation was assessed every 24 h. Data are presented as the mean±s.d. Results are from a representative experiment performed in triplicate. ( g ) Working model of Nedd8-mediated conjugation on the activation of Smurf1 ubiquitin ligase. Full size image The essential role of neddylation in the activation of Cullin-RING E3s has been extensively investigated. However, little is known about the role of neddylation in the regulation of HECT-type E3s. In this study, we demonstrate that Smurf1 is activated by neddylation. Smurf1 functions as an E3 ligase to promote its own autoneddylation. Smurf1 interacts with Nedd8 and Nedd8 E2 (Ubc12), and utilizes a distinct active site within the HECT N-lobe, that is, C426, to promote the transfer of Nedd8 for covalent conjugation. The autoneddylation of Smurf1 stimulates the activation of its ubiquitin E3 ligase and the degradation of substrates ( Fig. 8g ). In colorectal cancer tissues, Smurf1 is highly expressed and activated by neddylation, resulting in the promotion of cancer development. Our findings also demonstrate that both mammalian Smurf1 and yeast Rsp5 require neddylation to activate their ubiquitin ligase activity, suggesting that this mechanism is conserved across species. A previous proteomic analysis of Nedd8-associated proteins identified the HECT E3s UBR5/EDD1 and HUWE1/ARF-BP1 as potential Nedd8-interacting proteins [56] , suggesting that the regulatory role of Nedd8 on the activation of E3s might be broader than previously thought. This finding is consistent with the fact that neddylation is essential for the viability of most organisms and is involved in the development of various diseases, including cancer. Smurf1 and Rsp5 promote their own autoneddylation, primarily by acting as E3 ligases. In this regard, Smurf1 was shown to directly interact with Ubc12, and the binding motif pattern for this interaction is very similar to that of the neddylation co-E3 Dcn1. In the in vitro system, incubation with Nedd8, E1 and E2 was sufficient to promote Smurf1 neddylation, and this process was dependent on Smurf1 C426. We found that Smurf1 and Rsp5 represent a novel type of Nedd8 ligase, that is, thioester bond intermediate-type E3 ligases. As the currently reported Nedd8 ligases (that is, Dcn1, Roc1/Rbx1, IAPs, c-Cbl and MDM2) are all scaffold-type E3s [6] , [13] , [23] , [24] , [25] , [39] , [40] , [41] , [42] , our findings provide the first case of HECT-type of Nedd8 ligase and shed new light on the classification of Nedd8 ligases. In contrast to the huge number of ubiquitin ligases, <10 Nedd8 ligases have been identified. Our findings suggest that some HECT ubiquitin ligases might function as Nedd8 ligases. Smurf2, the close homologue of Smurf1, harbours >85% similarity with Smurf1 protein, implying that it might also function in the Smurf1-like manner. Seven other members of Nedd4 family are also worthy of further investigations. Smurf1 integrates ubiquitylation and neddylation pathways. Notably, C426 is critical for Smurf1 autoubiquitylation and Smurf1-mediated substrate ubiquitylation and degradation, whereas C699 is not required for Smurf1 autoneddylation, suggesting that the neddylation of Smurf1 precedes the ubiquitylation of Smurf1. The C426 neddylation active site of Smurf1 is located within the N-lobe large subdomain of HECT, while the C699 ubiquitylation active site is located within the C-lobe. These two sites are structurally close to each other. Future investigations are needed to elucidate whether any structural alterations occur when Nedd8 is conjugated to Smurf1. We tried our best to identify the neddylation sites of Smurf1. Through mass-spectrum analysis and biochemical mutation scanning, we found that Smurf1 was neddylated on multiple sites (at least six), including those located in the C2 domain, HECT domain and the WW-HECT linker. Smurf1 was predominantly mono-neddylated. Thus, the neddylation status is more complicated than the Cullins, which are usually mono-neddylated on a single lysine near the C terminus. Surprisingly, Rsp5, the yeast homologue of Smurf1, was mono-neddylated on a single site, K45. This is similar to the pattern of Cullins. In addition, Smurf1 harbours two catalytic cysteines for ubiquitylation and neddylation, whereas Rsp5 utilizes the same cysteine for the dual functions. So far, we have not exactly elucidated the mechanism of the differences. Although we demonstrated that Nedd8 regulates the protein levels of Smurf1 itself and Smurf1 substrates primarily through neddylation-promoted ubiquitylation, we cannot rule out other possibilities. For example, the NUB1 (Nedd8 ultimate buster-1), a Nedd8-interacting protein, can interacts with hRpn10/S5a subunit of 26S proteasome and function as an adaptor between Nedd8 and hRpn10. In this manner, NUB1 recruits Nedd8 and Nedd8-conjugated proteins to the proteasome for degradation independent of ubiquitylation [57] , [58] , [59] , [60] . Therefore, we cannot rule out the possibility that NUB1 and Nedd8 work together to downregulate the expression levels of Smurf1 and its substrates. We also demonstrated that the activation of Smurf1 by Nedd8 plays a crucial role in the progression of colorectal cancer. A large-scale immunohistochemical analysis of >300 colorectal cancer patient specimens revealed that Smurf1, Nedd8, Nedd8 E1 and Nedd8 E2 were significantly upregulated in cancer tissues compared with adjacent tissues, although the mechanisms that underlie this co-regulation remain unknown. Patients whose colorectal cancer featured high Smurf1 expression had especially poor prognosis. Thus, Smurf1 was not only elevated in its expression level but also in its ligase activity. Further studies in HCT116 cells and nude mice suggested that the autoneddylation of Smurf1 and the ubiquitin ligase activity of Smurf1 were critical for its tumour-promoting function. In contrast to the tumour-promoting role of Smurf1, Smurf2 has been suggested to function as a tumour suppressor gene since ablation of Smurf2 in mice resulted in increased susceptibility to various types of cancers in aged mice [61] . We noted that the NAE inhibitor MLN4924 has been recently identified as a novel approach to the treatment of acute myeloid leukaemia, head and neck cancer and liver cancer [62] , [63] , [64] . In addition, MLN4924 was demonstrated to inhibit tumour growth in lung cancer xenografts [65] . Therefore, our findings may have significant implications for the treatment of colorectal cancer. First, because of its ability to inhibit Smurf1 activity, MLN4924 might be a promising drug for colorectal cancer treatment. Second, small-molecule inhibitors of Smurf1 could be developed as novel anticancer agents. Taken together, this study identified neddylation as a critical activation mechanism for HECT-type ubiquitin ligases and also provided the first evidence of thioester bond-type Nedd8 ligase. These findings should contribute to deepen our understandings of the functions of the ubiquitin-like protein, Nedd8. Antibodies All antibodies were purchased as follows: anti-Smurf1 (ab117552, Abcam), anti-Ubc12 (ab56383, Abcam), anti-Smad5 (ab110022, Abcam), anti-Nedd8 (ALX-210-194-R200, Alexis Biochemicals), anti-Uba3 (PAB1774, Abnova), anti-Cul1 (AV03049, Sigma-Aldrich), anti-Roc1 (ab2977, Abcam), anti-NEDP1 (BS1475, Bioworld), anti-Smad4 (ab137861, Abcam), anti-Smad7 (SC-11392, Santa Cruz), anti-RhoA (ab68826, Abcam), anti-Myc, anti-GST, anti-His, anti-GAPDH (MBL), anti-Flag (Sigma-Aldrich) and mouse/rabbit IgG (Santa Cruz). Yeast two-hybrid screening Yeast two-hybrid screening was performed using the ProQuest two-hybrid system (Invitrogen). Briefly, the WW domains plus the HECT domain (amino acids 236–731) of human Smurf1 were cloned in-frame with the GAL4 DNA-binding domain in the vector pDBLeu to create pDBLeu-Smurf1-WH. MaV203 yeast cells were transformed with pDBLeu-Smurf1-WH and human liver cDNA library in pPC86 vector. A total of ~\n1 × 10 6 independent transformants were analysed, and clones were selected for positive interactions based on screening for expression of reporter genes His, LacZ and URA3. To eliminate interactions that originated from nonspecific promoter activation, we only considered DB-Smurf1-WH-AD-Prey pairs if they activated at least two out of three promoters. Positives were subsequently retested in fresh yeast cells, and their AD-Prey identities were determined by sequencing the corresponding PCR products. Co-immunoprecipitation assay Transfection was performed using Lipofectamine 2000 (Invitrogen). Cells were harvested 24–48 h after transfection and lysed in EBC lysis buffer (0.5% NP-40, 50 mM Tris, pH 7.6, 120 mM NaCl, 1 mM EDTA, 1 mM Na 3 VO 4 , 50 mM NaF and 1 mM β-mercaptoethanol) supplemented with protease inhibitor cocktail (Roche). For immunoprecipitation, 800 μg lysates were incubated with the appropriate antibody (1–2 μg) for 3–4 h at 4 °C followed by 1-h incubation with Protein A/G sepharose beads (GE Healthcare). The resulting immunoprecipitates were washed at least three times in NETN lysis buffer (150 mM NaCl, 1 mM EDTA, 50 mM Tris–HCl, pH 7.8, 1% NP-40, 1 mM phenylmethylsulfonyl fluoride, 0.5 μg ml −1 leupeptin and 0.5 μg ml −1 pepstatin) before being resolved by SDS-PAGE and immunoblotted with indicated antibodies. GST pull-down assay Ubc12 was inserted into thepGEX-6P-1 vector (Amersham). The Nedd8 sequence was inserted into the pGEX-4T-1 vector (Amersham) and fused with a 36-kDa thrombin protein upstream of the GST tag. The resulting construct expressed a thrombin-GST-Nedd8 protein of ~\n70 kDa. UbcH5c and UbcH7 were inserted into the pET-28a vector (Novagen). To detect the direct binding, bacteria-expressed GST-tagged proteins were immobilized on glutathione-Sepharose 4B beads (Amersham Biosciences) and then incubated with His-tagged proteins for 8 h at 4 °C under rotation. Beads were washed with GST-binding buffer (100 mM NaCl, 50 mM NaF, 2 mM EDTA, 1% NP-40 and protease inhibitor mixture) and proteins were eluted, followed by immunoblotting. Purify of His-tagged proteins using a Ni 2+ -NTA superflow cartridges The syringe was filled with Buffer NPI-10 (50 mM NaH 2 PO 4 , 300 mM NaCl, 10 mM imidazole, pH 8.0), and the cartridge equilibrated with 10 column volumes of buffer. The syringe was removed and filled with the neddylation reaction. The reaction was applied to the cartridge using the same flow rate. Using a fresh syringe and the same flow rate, the cartridge was washed with 10 column volumes of Buffer NPI-20 (50 mM NaH 2 PO 4 , 300 mM NaCl, 20 mM imidazole, pH 8.0). The protein was eluted from the cartridge with Buffer-NPI 250 (50 mM NaH 2 PO 4 , 300 mM NaCl, 250 mM imidazole, pH 8.0). In vivo modification assays To prepare cell lysates, cells were solubilized in modified lysis buffer (50 mM Tris, pH 7.4, 150 mM NaCl, 10% glycerol, 1 mM EDTA, 1 mM EGTA, 1% SDS, 1 mM Na 3 VO 4 , 1 mM DTT and 10 mM NaF) supplemented with a protease inhibitor cocktail. The cell lysate was incubated at 60 °C for 10 min. The lysate was then diluted 10 times with modified lysis buffer without SDS. The lysate was incubated with the indicated antibody for 3 h at 4 °C. Protein A/G-plus Agarose (Santa Cruz) was added, and the lysate was rotated gently for 8 h at 4 °C. The immunoprecipitates were washed at least three times in wash buffer (50 mM Tris, pH 7.4, 150 mM NaCl, 10% glycerol, 1 mM EDTA, 1 mM EGTA, 0.1% SDS, 1 mM DTT and 10 mM NaF). Proteins were recovered by boiling the beads in 2 × SDS sample buffer and analysed by western blot. Full images of key western blots are provided in Supplementary Fig. 11 . In vitro modification assays In vitro ubiquitylation and neddylation were performed using recombinant purified enzymes. His-Smurf1 was expressed in Escherichia coli BL21 (DE3). For the ubiquitylation assay, 0.7 μg of His-Smurf1 was incubated with 0.7 μg of E1, 1 μg of E2 (UbcH5c or UbcH7) and 15 μg of HA–ubiquitin (all from Boston Biochem) in 30 μl of ubiquitylation assay buffer (50 mM Tris–HCl, pH 8.0, 50 mM NaCl, 1 mMDTT, 5 mM MgCl 2 and 3 mM ATP). For the neddylation assay, 10 ng of His-Smurf1 was incubated with 2 μg of Nedd8, 10 ng of E1 (APPBP1-UBA3) and 200 ng of E2 (Ubc12) in a total reaction volume of 20 μl (40 mM Tris–HCl, pH 7.4, 5 mM MgCl 2 , 2 mM ATP and 2 mM DTT). Samples were incubated at 30 °C for 1 h, and reactions were terminated with 2 × SDS-PAGE loading buffer (20 mM Tris–HCl, pH 6.8, 100 mMDTT, 2% SDS, 20% glycerol and 0.016% Bromophenol blue) before western blotting. If needed, the neddylation reaction sample was first purified with Ni 2+ -NTA Superflow Cartridges (QIAGEN). In vitro thioester bond assay All in vitro Nedd8 thioester and Ub thioester assays were carried out in 15 μl reaction buffer (50 mM Tris (pH 7.5), 10 mM MgCl 2 and supplemented with 3 mM ATP; 5 × 15 μl reactions where incubation times, protein concentrations or SDS-PAGE buffer (±DTT(100 mM)) were varied using E1 (APPBP1-UBA3or Ube1) and E2 (Ubc12 or UbcH5c), Nedd8 or Ub (all from Boston Biochem), and 1 mM His-Smurf1or the mutations. Reactions were incubated at room temperature for 5 min (Nedd8 thioester) or 10 min (Ub thioester assays) and stopped with E1 stop buffer. Nedd8 thioester or Ub thioester were detected using Smurf1 antibody. RNA interference The sequences of the used siRNAs are listed below. Nedd8, 1#: 5′-AGCGAAUCAAGGAGCGUGUTT-3′, 2#: 5′-GUGGUUCAGUCCUUCACCUTT-3′, 3#: 5′-CAGCAGCYGAUUACAAGAUTT-3′, the non-targeting siRNA, 5′-UUCUCCGAACGUGUCACGUTT-3′. These siRNAs were synthesized by Shanghai GenePharm and transfected using Lipofectamine RNAi MAX (Invitrogen). siRNAs of Ubc12, UbcH5c, Uba3 and Roc1 were purchased from Dharmacon, and 100 nM siRNA was transfected into cells with Dharma FECT. For establishment of stably Smurf1-depleted HCT116 cell lines, the lentivirus-mediated Smurf1 shRNA sequence is 1#: 5′-GGTTACACCACATCATGAA-3′; 2#: 5′-CTCAACCGACACTGTGAAA-3 and the control sequence 5′-TGCGTTGCTAGTACCAAC-3′. The targeting sequences were cloned into pGCSIL-PUR vector (Shanghai GeneChem). The depletion efficiency was evaluated by western blot analysis. Yeast strains and plasmids All yeast strains used in this study are derivatives of DF5 alpha haploid (his3-Δ200, leu2-3, 2-112, lys2-801, trp1-1 (am) and ura3-52). The Rub1-, Ula1-, Uba3- and Ubc12-knockout strains and the Rsp5 temperature-sensitive strain (rsp5Δ::HIS3; ura3-52::rsp5-2::URA3) have been previously described [66] . The wild-type and C-terminal GG-deleted versions of the Rub1 expression plasmid and the HA-Nedd8 plasmid have been previously described [66] . Wild-type and K-to-A mutations of Rsp5 fragments were inserted into the p413 ADH promoter expression vector with an HA tag fused at the N terminus. The information about Flag-Rub1 and HA-Rub1 strains are: Flag-Rub1 was constructed in yeast centromeric vector YCplac2 under control of ADH promoter except in Fig. 7f where the endogenous promoter of Rub1 was used. HA-Rub1 was constructed in yeast integrating vector YIplac204 under control of ADH promoter. To demonstrate that Rsp5 is neddylated on that lysine without Nedd8 overexpression, we constructed endogenous expression of Rub1 to show Rsp5 could be modified under endogenous level of Rub1. Briefly, endogenous promoter of Rub1 (500 bp upstream of Rub1 ORF) following Flag-tagged Rub1 ORF and Rub1 terminator (360 bp downstream of Rub1 ORF) was constructed into yeast centromeric vector YCplac22. Yeast cell immunoprecipitation Yeast cells from YPD cultures of different haploid strains were collected and suspended in PBS buffer containing 10% glycerol, 10 mM NEM, 20 mM IAA and protease inhibitor cocktail (Roche). Cells were lysed by sonication, and the lysates were centrifuged at 5,000 g for 10 min. Supernatants were collected for further immunoprecipitation with antibody-coupled protein A–Sepharose and eluted in SDS-loading buffer. Patients and tissue specimens The colorectal cancer tumour specimens used in the tissue microarray (TMA) studies were obtained from a tissue bank maintained in the Zhongshan Hospital at Fudan University. The patients underwent surgical resection between 2004 and 2011. For each patient, the diagnosis of colorectal cancer was confirmed by pathologic examination. All tumours were primary and untreated before surgery, and clinical pathological information for the tumours, including histological grade, TNM stage classification and immunohistochemical staining for Smurf1, Nedd8, NAE1 and Ubc12, was available. Tumours were staged according to the TNM classification system of the International Union against Cancer (edition 7). Tumour size was measured and converted to tumour volume (TV) according to the following formula: TV (mm 3 )=( a × b 2 )/2, where a and b are the largest and smallest diameters, respectively. Vascular invasion was determined by microscopic examination of the resected specimen. Approval for this study was obtained from the Zhongshan Hospital Research Ethics Committee. Informed consent was obtained from all subjects or their relatives. Immunohistochemical staining We performed immunohistochemical (IHC) staining for Smurf1, Nedd8, NAE1, Ubc12 and NEDP1 on the same paraffin-embedded tissue blocks that were used for clinical diagnosis. Immunohistochemistry was performed using the avidin–biotin complex method (Vector Laboratories), including heat-induced antigen-retrieval procedures. Incubation with polyclonal antibodies against Smurf1 (H60; 1:50 dilution; Santa Cruz), Nedd8 (LS-C118606; 1:100; LifeSpan BioSciences), NAE1 (LS-C100844; 1:50; LifeSpan BioSciences), Ubc12 (LS-C138461; 1:100; LifeSpanBioSciences) and NEDP1 (BS1475; 1:50; Bioworld) was performed at 4 °C for 18 h. Quality assessment was performed on each batch of slides by including a negative control in which the primary antibody was replaced by 10% normal goat serum to preclude non-specific signals. Staining was assessed by pathologists who were blinded to the sample origins and the patient outcomes. The widely accepted German semi-quantitative scoring system was used to score staining intensity and extent in different areas. Each specimen was assigned a score according to the intensity of the nucleic, cytoplasmic and membrane staining (no staining=0; weak staining=1, moderate staining=2 and strong staining=3) and the extent of stained cells (0–5%=0, 5–25%=1, 26–50%=2, 51–75%=3 and 76–100%=4). The final immunoreactivity score was determined by multiplying the intensity score by the score for the extent of stained cells, generating a score that ranged from 0 (the minimum score) to 12 (the maximum score). Tissue microarray After screening haematoxylin and eosin-stained slides for optimal tumour content, we constructed TMA slides (Shanghai Biochip Company, Ltd., Shanghai, China). Two cores of tissue were collected from non-necrotic areas of tumour foci and from peritumoral tissue adjacent to the tumour. To assess the possibility that positive expression reflected a direct effect of the tumours, we took peritumoral tissue within 10 mm. Punch cores with the longest dimension of 1.0 mm were used. TMA sections with 458 pairs of intratumoral and matched peritumoral samples were constructed. Sections (4 μm) of the resulting TMA blocks were prepared using standard techniques. Tumour growth in mice The experimental procedures in mice have been approved by the Animal Care and Use Committee of Academy of Military and Medical Sciences. BALB/c nude mice (6-week old, 18.0±2.0 g) were obtained from Shanghai Laboratory Animal Center (SLAC, China). HCT116 cells (5 × 10 6 per mouse) were inoculated subcutaneously into the right flank of the mice. Tumour size was measured every 3 days and converted to TV according to the following formula: TV (mm 3 )=( a × b 2 )/2, where a and b are the largest and smallest diameters, respectively. All animals were killed 5 weeks after injection, and the transplanted tumours were removed, weighed and fixed for further study. Real-Time PCR For mRNA analysis, total RNA was isolated by Trizol, and was converted to cDNA using the superscript III First Strand Synthesis System (Invitrogen). Quantitative PCR was performed using the Bio-Rad IQ5 System (Bio-Rad). PCR reactions were carried out in 25 μl reactions using SYBR Green PCR master mix (Bio-Rad) and 0.2 μM specific primers. Primer sequences for specific genes are described in Supplementary Table 2 . Cell proliferation assay Smurf1 WT or C426A, C530A, C699A mutant was each stably transfected into HCT116 cells that were depleted of Smurf1 with Lentivirus-coupled shRNA against Smurf1. Synonymous mutations were made in these Smurf1 expression constructs to avoid the interference between the overexpression and depletion system. The colorectal cancer HCT116 cells were plated on 96-well plates (1,000 cells per well). The plates were incubated at 37 °C. Cell growth was analysed using Cell Titer 96-Aqueous assay kit (Promega) according to the manufacturer’s directions. Cell numbers were estimated every 24 h by adding MTS to the wells 1 h before absorbance at 490 nm was measured. Each cell line was set up in 4 replicate wells, and the experiment was repeated thrice. Each data point represents a mean±s.d. Cell migration assay Cell migration assay was performed in 24-well transwell plate with 8-μm polyethylene terephalate membrane filters (Falcon cell culture insert (Becton–Dickinson)) separating the lower and upper culture chambers. In brief, HCT116 cells were plated in the upper chamber at 5 × 10 4 cells per well in serum-free DMEM medium. The bottom chamber contained DMEM with 10% FBS. Cells were allowed to migrate for 18 h in a humidified chamber at 37 °C with 5% CO 2 . After the incubation period, the filter was removed and non-migrant cells on the upper side of the filter were detached using a cotton swab. Filters were fixed with 4% formaldehyde for 15 min and cells located in the lower filter were stained with 0.1% crystal violet for 20 min and photographed. Statistical analysis Statistical analyses were performed using IBM SPSS 19.0 software. The χ 2 test was used to compare qualitative variables. The expression of proteins in colorectal cancer tumours and matched adjacent tissue was compared using the Wilcoxon test. Correlations between Smurf1 expression and Nedd8, NAE1 and Ubc12 expression were determined using Pearson’s correlation test. Score comparisons between groups were assessed using the Kruskal–Wallis test. We defined cumulative survival as the time from the date of diagnosis to the date of the patient’s death from colorectal cancer. Cumulative survival curves were computed using the Kaplan–Meier method and compared between groups using the log-rank test. All statistical tests were two-sided, and P -values <0.05 were considered statistically significant. How to cite this article: Xie, P. et al . The covalent modifier Nedd8 is critical for the activation of Smurf1 ubiquitin ligase in tumorigenesis. Nat. Commun. 5:3733 doi: 10.1038/ncomms4733 (2014).